Photobiocatalytic chemistry of oxidoreductases using water as the electron donor To date, water has been poorly studied as the sacrificial electron donor for biocatalytic redox reactions using isolated enzymes. Here we demonstrate that water can also be turned into a sacrificial electron donor to promote biocatalytic redox reactions. The thermodynamic driving force required for water oxidation is obtained from UV and visible light by means of simple titanium dioxide-based photocatalysts. The electrons liberated in this process are delivered to an oxidoreductase by simple flavin redox mediators. Overall, the feasibility of photobiocatalytic, water-driven bioredox reactions is demonstrated. Biocatalysts are gaining ground as competitive tools for organic chemistry [1] , [2] , [3] , [4] , [5] , [6] , [7] , [8] . Their high selectivity enables shorter and more efficient synthetic routes and bears the promise for greener chemistry. Today, hydrolytic enzymes are well-established on industrial scale and oxidoreductases are ready to follow. This latter class of enzymes catalyses a broad range of synthetically useful transformations ranging from (enantio)selective reduction and oxidations to specific oxyfunctionalization or halogenation [9] . Some oxidoreductases, such as dehydrogenases, are, however, cofactor-dependent enzymes, which represents a major drawback for practical applications. Usually, the required reductants (either for reduction of the substrate or reductive activation of molecular oxygen to perform oxyfunctionalisation chemistry) are delivered via natural electron transport chains. These electron transport chains often comprise several enzymes and cofactors to connect the oxidoreductases to the reduced nicotinamide cofactors NADH (β-nicotinamide adenine dinucleotide) or NADPH (β-nicotinamide adenine dinucleotide phosphate). The latter themselves are rather costly necessitating an enzymatic regeneration system to allow for their use in catalytic quantities. Today, a broad range of such regeneration systems are available, in principle solving this cofactor challenge [10] , [11] , [12] , [13] . The resulting multi-enzyme cascades ( Fig. 1 ) comprise up to two extra enzymes and cofactors in addition to the actual production enzyme. 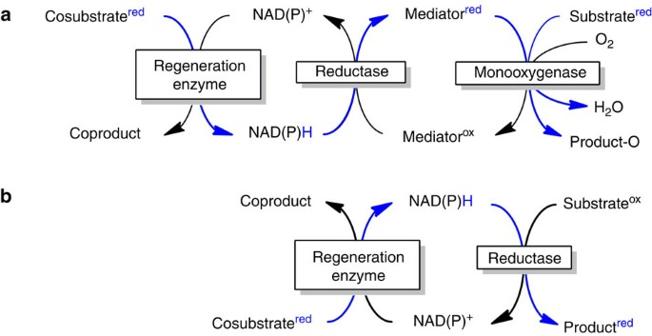Figure 1: Schematics of electron transport chains. Representation of the traditional electron transport chain to supply monooxygenases (a) and reductases (for example, alcohol dehydrogenases or old yellow enzymes) (b) with reducing equivalents. In both cases, a high-energy content cosubstrate is oxidized by a regeneration enzyme thereby regenerating the reduced nicotinamide cofactor (NADH or NADPH). The latter delivers two electrons either directly to the production enzyme (for example, alcohol dehydrogenases, old yellow enzymes but also some monooxygenases) or (as in case of many monooxygenases) indirectly via an electron mediator system (such as flavins or FeS-proteins). The flow of electrons is shown in blue. Typical examples for regeneration enzymes comprise formate dehydrogenase, alcohol dehydrogenase, glucose dehydrogenase and so on oxidizing the respective cosubstrates such as formic acid, ethanol/isopropanol or glucose. Figure 1: Schematics of electron transport chains. Representation of the traditional electron transport chain to supply monooxygenases ( a ) and reductases (for example, alcohol dehydrogenases or old yellow enzymes) ( b ) with reducing equivalents. In both cases, a high-energy content cosubstrate is oxidized by a regeneration enzyme thereby regenerating the reduced nicotinamide cofactor (NADH or NADPH). The latter delivers two electrons either directly to the production enzyme (for example, alcohol dehydrogenases, old yellow enzymes but also some monooxygenases) or (as in case of many monooxygenases) indirectly via an electron mediator system (such as flavins or FeS-proteins). The flow of electrons is shown in blue. Typical examples for regeneration enzymes comprise formate dehydrogenase, alcohol dehydrogenase, glucose dehydrogenase and so on oxidizing the respective cosubstrates such as formic acid, ethanol/isopropanol or glucose. Full size image Clearly, such complicated electron transport chains are difficult to optimize and lack robustness required for a chemical transformation at scale. This also gives an explanation why cofactor-dependent oxidoreductases (such as dehydrogenases or monooxygenases) are lagging behind ‘simple’ cofactor-independent enzymes (such as hydrolases, oxidases and even peroxidases) with respect to their implementation in preparative organic chemistry. A more elegant approach is to deliver the reducing equivalents directly from the cosubstrate to the oxidoreductases, thereby shortcutting the complicated natural electron transport chain. Ever since the pioneering work by Vilker and coworkers [14] , a range of direct regeneration approaches have been reported [15] , [16] , [17] , [18] , [19] , [20] , [21] , [22] , [23] , [24] , [25] , [26] , [27] , [28] . Another issue is the fact that the majority of cosubstrates are valuable compounds themselves as they are generally highly reduced compounds, which, when applied for cofactor regeneration, are wasted as simple electron donors and generate additional (waste) by-products. Indeed, water would be the most attractive sacrificial electron donor but its high stability and very low oxidation potential require additional energy input to activate water as electron donor. Nature’s answer to this challenge is photosynthesis where visible light is used as thermodynamic driving force to promote water oxidation leading to the formation of molecular oxygen and biogenic reducing equivalents in form of reduced nicotinamide cofactors (NAD(P)H). Natural photosynthesis, however, is challenging to apply in vitro , mainly due to stability issues [29] , [30] , [31] . Nevertheless, photosynthesis has inspired chemists to search for robust (inorganic) photocatalysts capable of mimicking the natural process [32] . A great variety of potentially useful photocatalysts have resulted from the ongoing research on the conversion of solar energy into chemical energy [33] , [34] . Light-driven water splitting is a particular focus of research, resulting in many elegant biomimetic photocatalytic systems, with titanium dioxide being the most widely used photocatalyst [35] . TiO 2 doped with noble metals and non-metal elements, such as N, C and S, have also been extensively studied. However, to the best of our knowledge, utilization of these reducing equivalents to promote (bio)catalytic redox reactions has not been reported yet. It is however worth mentioning here that TiO 2 -generated H 2 O 2 has been used to promote peroxidase-catalysis in biosensor applications [36] , [37] , [38] . Here we use light-driven and TiO 2 -promoted water oxidation to drive biocatalytic redox reactions. As a model transformation, we have chosen the stereospecific reduction of conjugated C=C-double bonds catalysed by old yellow enzymes. The feasibility of this photoenzymatic reaction scheme is demonstrated. Photobiocatalytic reduction reactions To demonstrate the feasibility of the envisaged combination of photocatalytic water oxidation and enzymatic redox reactions, we chose the asymmetric reduction of conjugated C=C-double bonds as a model reaction ( Fig. 2 ). As photocatalyst, a system formed by gold nanoparticles deposited on TiO 2 , reported as an active catalyst for the photochemical water splitting reaction [39] , was chosen. The model biocatalyst was the old yellow enzyme homologue from Thermus scotoductus SA-01 ( Ts OYE) [40] , [41] , catalysing the stereoselective trans -hydrogenation of Ketoisophorone ( 1 ) to ( R )-Levodione ( 2 ) ( Fig. 2 ). Flavin mononucleotide (FMN) played a dual role as an enzyme prosthetic group and (photoexcitable) redox mediator delivering electrons from the photocatalyst to the enzyme. 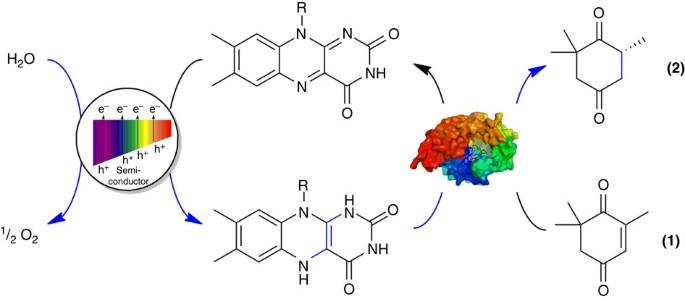Figure 2: The proposed photobiocatalytic reduction system. TiO2-based photocatalysts mediate the light-driven oxidation of water yielding O2as sole by-product. The reducing equivalents liberated are transferred via flavin mediation to the active site of the oxidoreductase (here: the old yellow enzyme homologue fromThermus scotoductusSA-01). Figure 2: The proposed photobiocatalytic reduction system. TiO 2 -based photocatalysts mediate the light-driven oxidation of water yielding O 2 as sole by-product. The reducing equivalents liberated are transferred via flavin mediation to the active site of the oxidoreductase (here: the old yellow enzyme homologue from Thermus scotoductus SA-01). Full size image Upon irradiating the catalytic components indicated in Fig. 2 : Au-TiO 2 (10 gl −1 ), FMN (200 μM) and Ts OYE (15.2 μM) with UV light (Hg-doped Xe-lamp, 200 W) at 50 °C we were pleased to observe conversion of Ketoisophorone ( 1 ) (10 mM) into ( R )-Levodione ( 2 ) (66% conversion, 86% ee after 6 h). If the reaction was carried out in the dark and in the presence of H 2 only, 26% conversion and racemic product was obtained indicating that the cofactor is reduced as suggested in Fig. 2 and not (or only to a minor extent) by molecular H 2 . It is also worth mentioning that using stoichiometric amounts of NADPH (in the darkness under otherwise identical conditions) resulted in significantly lower yield (49% as compared with 66%). This may unambiguously be explained by the aerobic reaction conditions. Flavoproteins are known to be reoxidized in the presence of molecular oxygen. This competing uncoupling of the flavin reduction from substrate reduction was not compensated in the presence of stoichiometric amounts of NADPH, whereas the photocatalytic approach continuously provided Ts OYE with reducing equivalents. To prove that indeed water serves as sacrificial electron donor, qualitative experiments were carried out using labelled water (H 2 18 O) as reaction medium under standard reaction conditions. Gratifyingly, 18 O 2 could be identified by GC/MS in the gas phase, thus strongly supporting our initial hypothesis. The high enantiomeric purity of the product suggested a biocatalytic reduction reaction by Ts OYE and FMN. However, also direct reduction of Ketoisophorone ( 1 ) at the photocatalyst surface (Au-TiO 2 ) and/or by free reduced FMN (FMNH 2 ) may occur. Indeed, performing the experiment described above in the absence of Ts OYE and FMN gave essentially identical conversion but formed the racemic product. Overall, these results suggest that Au-TiO 2 -catalysed oxidation of water was the overall rate-limiting step in the photoenzymatic reduction of Ketoisophorone ( 1 ). Kinetic studies Aiming at further understanding of the catalytic mechanism, we performed a range of experiments systematically varying the catalysts concentrations. Particularly, we aimed at understanding the apparent competition between Ts OYE-catalysed and non-enzymatic reduction of Ketoisophorone ( Fig. 3 ). 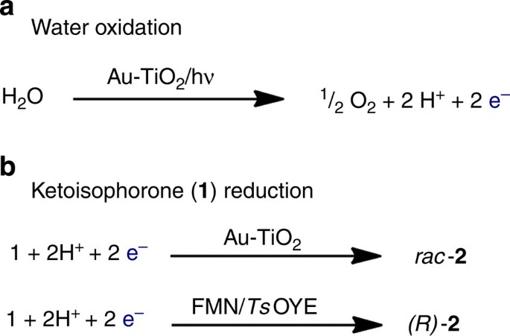Figure 3: Proposed elementary steps of the photoenzymatic reduction of Ketoisophorone. (a) The photocatalyst (Au-TiO2) oxidises water yielding O2and electrons in the valence band of the photocatalyst. (b) These electrons can be transferred to the substrate directly (non-enzymatic step, yielding racemic product) or via FMNH2to the enzyme (resulting in enantiomerically pure product). Figure 3: Proposed elementary steps of the photoenzymatic reduction of Ketoisophorone. ( a ) The photocatalyst (Au-TiO 2 ) oxidises water yielding O 2 and electrons in the valence band of the photocatalyst. ( b ) These electrons can be transferred to the substrate directly (non-enzymatic step, yielding racemic product) or via FMNH 2 to the enzyme (resulting in enantiomerically pure product). Full size image In a first set of experiments, we varied the concentration of photocatalyst under otherwise identical conditions. As shown in Fig. 4 , the initial rate of the overall reaction directly depended on the photocatalyst concentration applied. The individual time courses are given in the Supplementary Fig. 1 . The apparent saturation kinetics (leveling off of the curve at high photocatalyst concentrations) may be explained by the decreasing optical transparency of the reaction medium leading to suboptimal illumination of the TiO 2 -particles. Alternatively, this saturation behaviour may indicate Michaelis–Menten-type saturation of the enzyme with FMNH 2 as ‘cosubstrate’ However, the formal specific activity of Ts OYE determined at the highest TiO 2 concentration applied in Fig. 4 corresponds to 0.1 U mg −1 , which is somewhat lower than the reported activity (albeit under optimized reaction conditions) [40] , [41] , indicating that the full catalytic potential of Ts OYE is not fully exploited here ( vide infra ). Varying the biocatalyst concentration, however, had no significant influence on the initial rate of the reaction ( Fig. 5 ). We like to interpret these observations as the photocatalytic water oxidation reaction being overall rate limiting. Still, the enzyme concentration had a marked influence on the optical purity of the Levodione ( 2 ) product. As shown in Fig. 5 , racemic product was formed in the absence of Ts OYE, whereas, already in the presence of relatively small concentrations of the enzyme, significant optical purities were observed. At, saturation concentrations’ the optical purities observed (94% ee) were essentially identical to those observed under natural conditions [40] , [41] . Hence, we conclude that the reducing equivalents provided by the photocatalyst are more efficiently used by the biocatalyst (leading to highly enantiomerically pure product) than for spontaneous chemical reduction. 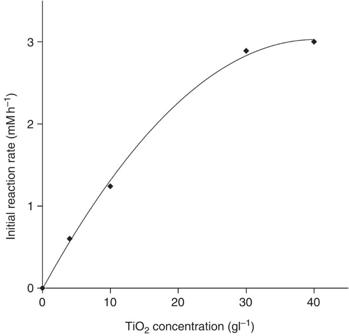Figure 4: Effects of photocatalyst concentration. Influence of the photocatalyst concentration on the initial rate of the photoenzymatic reduction of Ketoisophorone. Reaction conditions: 2.5 ml buffer (50 mM MOPS, pH 7.5, 10 mM CaCl2) containing 10 mM Ketoisophorone; 200 μM FMN; 20 mg lyophilizedTsOYE preparation (15.2 μMTsOYE); 323 K. Figure 4: Effects of photocatalyst concentration. Influence of the photocatalyst concentration on the initial rate of the photoenzymatic reduction of Ketoisophorone. 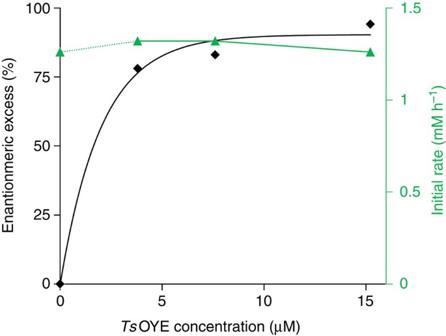Figure 5: Effects of biocatalyst concentration. Influence of the biocatalyst concentration on initial rate (green triangle) and enantioselectivity (black diamond) of the photoenzymatic reduction of Ketoisophorone. Reaction conditions: 2.5 ml buffer (50 mM MOPS, pH 7.5, 10 mM CaCl2) containing 10 mM Ketoisophorone; 200 μM FMN lyophilizedTsOYE preparation; 10 gl−1Au-TiO2; 323 K. Reaction without enzyme: 2.5 ml buffer (50 mM MOPS, pH 7.5, 10 mM CaCl2) containing 10 mM ketoisophorone. Reaction conditions: 2.5 ml buffer (50 mM MOPS, pH 7.5, 10 mM CaCl 2 ) containing 10 mM Ketoisophorone; 200 μM FMN; 20 mg lyophilized Ts OYE preparation (15.2 μM Ts OYE); 323 K. Full size image Figure 5: Effects of biocatalyst concentration. Influence of the biocatalyst concentration on initial rate (green triangle) and enantioselectivity (black diamond) of the photoenzymatic reduction of Ketoisophorone. Reaction conditions: 2.5 ml buffer (50 mM MOPS, pH 7.5, 10 mM CaCl 2 ) containing 10 mM Ketoisophorone; 200 μM FMN lyophilized Ts OYE preparation; 10 gl −1 Au-TiO 2 ; 323 K. Reaction without enzyme: 2.5 ml buffer (50 mM MOPS, pH 7.5, 10 mM CaCl 2 ) containing 10 mM ketoisophorone. Full size image It is worth mentioning that the photocatalyst could be reused at least twice without appreciable activity reduction ( Supplementary Fig. 2 ). Towards visible light-driven reactions As mentioned above, the Au-TiO 2 -catalysed oxidation of water appeared to be the overall rate-limiting step. Therefore, we hypothesized that other dopants such as transition metal oxides easily changing their valence might be more efficient water oxidation catalysts. In this respect, V(V) oxide may be a suitable cocatalyst since V 5+ can coordinate water to form hydroxyl radicals bonded to the vanadium and thereby catalyse water oxidation. In fact, substituting the previously used Au-TiO 2 by V-TiO 2 resulted in a significantly increased overall reaction rate (more than two times faster under otherwise identical conditions) and resulted in full conversion of the starting material into ( R )-Levodione ( 2 ) at slightly decreased optical purity of the product (80% ee). Again, control experiments in the absence of the biocatalyst resulted in comparable yields albeit forming racemic product, while no product formation was observed in the dark (in the presence and absence of H 2 ). Representative progression curves for Au-TiO 2 - and V-TiO 2 -catalysed water oxidation to promote Ts OYE-catalysed reduction reactions are shown in Fig. 6 . 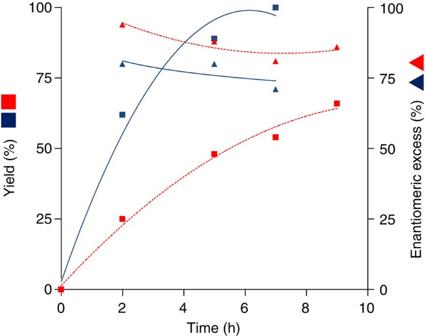Figure 6: Time courses of reactions. Comparison of the time courses of Au-TiO2(red symbols) and V-TiO2(blue symbols)-driven reductions of Ketoisophorone with respect to yield (squares) and optical purity of the product (triangles) Reaction conditions: 2.5 ml buffer (50 mM MOPS, pH 7.5, 10 mM CaCl2) containing 10 mM Ketoisophorone; 200 μM FMN; 15.2 μMTsOYE); 10 gl−1photocatalyst; 323 K. Figure 6: Time courses of reactions. Comparison of the time courses of Au-TiO 2 (red symbols) and V-TiO 2 (blue symbols)-driven reductions of Ketoisophorone with respect to yield (squares) and optical purity of the product (triangles) Reaction conditions: 2.5 ml buffer (50 mM MOPS, pH 7.5, 10 mM CaCl 2 ) containing 10 mM Ketoisophorone; 200 μM FMN; 15.2 μM Ts OYE); 10 gl −1 photocatalyst; 323 K. Full size image Even more interestingly about V-TiO 2 is its water oxidation activity in the visible-light range. Ideally, photoredox biocatalytic reactions would be performed under sunlight irradiation. Therefore, we also investigated V-TiO 2 as regeneration catalyst for Ts OYE in the presence of visible light using polychromatic light of wavelengths longer than 385 nm under otherwise identical conditions to the experiments reported before. Under these conditions, very promising results of more than 50% yield of Levodione (at optical purities greater than 85% ee) were obtained within 9 h reaction time. With this proof-of-concept study, we have demonstrated for the first time that catalytic water oxidation mediated by robust TiO 2 semiconductors can be productively coupled to oxidoreductases achieving photobiocatalytic redox reactions. Thereby, two emerging technologies with great potential for the chemistry of the 21st century have been successfully combined to create a new, promising discipline of Green Chemistry. Admittedly, the technology is in its infancy, but further mechanistic studies will reveal optimal reaction conditions and expand this concept to other biocatalytic redox transformations. We are convinced that the concept introduced here will significantly have an impact on redox biocatalysis. Materials Ketoisophorone, FMN, HAuCl 4 , Calcium Chloride and MOPS were purchased from Sigma-Aldrich; Aeroxide TiO 2 P 25 was purchased from Degussa (Evonik). Photocatalyst preparation Au-TiO 2 (1% Au) and V-TiO 2 (1% V) were prepared according to literature procedures [39] , [42] . An exemplary TEM picture of the photocatalyst preparation is shown in Supplementary Fig. 3 . Enzyme production Ts OYE was purified according to a previously published procedure [41] . Escherichia coli BL21 (DE3) harbouring a pET22b(+) plasmid containing the gene encoding for Ts OYE was cultivated in minimal medium at 30 °C. Upon reaching an OD 600 of 0.45, Ts OYE expression was induced by the addition of 0.1 mM final IPTG (isopropyl β- D -1-thiogalactopyranoside) followed by further cultivation for 12 h. The cell pellet (resulting from centrifugation and washing with 20 mM MOPS buffer pH 7.5 containing 5 mM CaCl 2 ) was suspended in fresh washing buffer. Cell disruption was achieved by two passages through the French press followed by heat treatment at 70 °C for 1.5 h. After centrifugation, to remove insoluble cell debris and denaturated proteins, a bright yellow solution of Ts OYE (more than 95% pure as estimated by SDS-page analysis) was obtained. For storage, this solution was freeze dried and remained more than 90% of its original activity upon storage at 4°C for at least several months. Standard reaction The photoreactor was a cylindrical quartz vessel (Vicilab®) (48 ml total volume). A typical reaction was performed as follows: 25 mg Au-TiO 2 (1%Au) or V-TiO 2 (1% V); 200 μM FMN and 10 mM CaCl 2 were added sequentially to 2 ml MOPS buffer pH 7. The whole system was purged with an argon flow for at least 30 min before irradiation to ensure the absence of oxygen in the system. Afterwards, ketoisophorone (10 mM final concentration) and 20 mg of lyophilized Ts OYE dissolved in 500 μl MOPS buffer were added with a syringe to the reaction mixture. The system was heated until 323 K. Then, it was irradiated for certain time using 200 W Xenon-doped mercury lamp (Hamamatsu Lightningcure LC8, spot light source L9566-04; DB 4719 input 100–240 V 300 VA 50–60 Hz), without filter, 1 cm distance. For visible light experiment, the output of 200 W Xenon-doped mercury lamp was filtered thought a cutoff filter ( λ >380 nm). GC analyses were performed with a HP-5 column (30 m × 0.320 mm) from Agilent technologies. The amount of product was quantified from the peak areas using an external standard methodology. Reduction reaction by H 2 The reaction was carried out as follows: a mixture of 12.5 mg Au-TiO 2 (1%Au) or V-TiO 2 (1% V), Ketoisophorone (10 mM final concentration) were added sequentially to 1.25 ml MOPS buffer pH 7. The resultant suspension was bubbled with H 2 during 10 min, afterwards the autoclave was pressurized until 5 bars of H 2 .The system was heated at 323 K and kept it under vigorous stirring. GC analyses were performed with a HP-5 column (30 m × 0.320 mm) from Agilent technologies. The amount of product was quantified from the peak areas using an external standard methodology. H 2 18 O experiment The photoreactor was a cylindrical quartz vessel (Vicilab) (48 ml total volume) with an inlet and outlet with independent valves and equipped with a manometer to determine the pressure. The reaction was performed as follows: 12.5 mg V-TiO 2 (1% V); 200 μM FMN; 10 mM CaCl 2 and 10 mg of lyophilized Ts OYE were added sequentially to 1 ml MOPS buffer pH 7 prepared with H 2 18 O. The whole system was purged with an argon flow for at least 30 min before irradiation to ensure the absence of oxygen in the system. Afterwards, ketoisophorone (10 mM final concentration) was added with a syringe to the reaction mixture. The system was heated until 323 K. Then, it was irradiated for certain time using 200 W Xenon-doped mercury lamp (Hamamatsu Lightningcure LC8), 1 cm distance. 18 O 2 evolved in course of the reaction was detected by GC/MS. How to cite this article: Mifsud, M. et al . Photobiocatalytic chemistry of oxidoreductases using water as the electron donor. Nat. Commun. 5:3145 doi: 10.1038/ncomms4145 (2014).